Heat-shock protein dysregulation is associated with functional and pathological TDP-43 aggregation Conformational disorders are involved in various neurodegenerative diseases. Reactive oxygen species (ROS) are the major contributors to neurodegenerative disease; however, ROS that affect the structural changes in misfolded disease proteins have yet to be well characterized. Here we demonstrate that the intrinsic propensity of TDP-43 to aggregate drives the assembly of TDP-43-positive stress granules and soluble toxic TDP-43 oligomers in response to a ROS insult via a disulfide crosslinking-independent mechanism. Notably, ROS-induced TDP-43 protein assembly correlates with the dynamics of certain TDP-43-associated chaperones. The heat-shock protein (HSP)-90 inhibitor 17-AAG prevents ROS-induced TDP-43 aggregation, alters the type of TDP-43 multimers and reduces the severity of pathological TDP-43 inclusions. In summary, our study suggests that a common mechanism could be involved in the pathogenesis of conformational diseases that result from HSP dysregulation. Oxidative damage, which is caused by impaired mitochondrial respiratory function [1] , [2] , is associated with a progressive decline in neuronal functioning and is one of the most important causes of neurodegenerative and age-associated diseases. Elevated levels of intracellular reactive oxygen species (ROS), which can be induced by hydrogen peroxide (H 2 O 2 ) treatment or deficiencies in superoxide dismutase (SOD1) or sirtuins, induce premature senescence and reduce cellular life spans [3] , [4] . During the natural progression of neurodegenerative diseases, ROS insults have been suggested to occur at two stages, the pre-symptom stage and the post-inclusion accumulation stage [5] . The distribution of subsequent oxidation products, such as 8-hydroxyguanosine and nitrotyrosine, and the areas of the brain that are affected by Alzheimer’s disease (AD) are strongly correlated, supporting the hypothesis that local increases in ROS activity in certain brain regions contribute to AD [6] , [7] , [8] . In addition, the reduced expression of proteins involved in nuclear import, including susceptibility protein and importin-α2, has been observed post mortem in the brains of individuals with sporadic amyotrophic lateral sclerosis (ALS) and has been linked to the ROS-induced inhibition of nuclear import [9] . Recently, TAR DNA-binding protein 43 (TDP-43) oxidation has been observed in a type of frontotemporal lobe degeneration that is characterized by ubiquitin-positive inclusion (FTLD-U) pathology, in which the inclusions are possibly formed by intra- and inter-disulfide crosslinking [10] . Several studies have suggested that once ROS production begins, oxidized TDP-43 polymerizes and is recruited into stress granules (SGs) [10] , [11] , [12] . These TDP-43-positive SGs are often observed in patients with various types of neurological diseases, including FTLD-U, ALS, AD and brain injury, and have been linked to early pathogenesis [10] . These data support a common pathological role for ROS in neurodegenerative disease. TDP-43 is a multifunctional protein that promotes exon 9 skipping in cystic fibrosis transmembrane conductance regulator mRNA by binding to the UG repeat motifs at the 3′ splice site; TDP-43 might regulate nuclear subdomains, translation and microRNA biogenesis [13] , [14] . The loss of TDP-43 results in large-scale pre-mRNA mis-splicing and increased neuronal vulnerability [15] . TDP-43 has been identified as an FTLD-U- and ALS-associated gene, and disease-associated mutations in its C-terminus cause neuronal dysfunction and loss [16] . The TDP-43 C-terminus is prone to spontaneous aggregation, and pathological TDP-43 aggregates from diseased brains can function as seeds to induce seed-dependent TDP-43 aggregation in cells [17] . Recently, we demonstrated that a GQN-rich domain in the non-amyloid disease protein TDP-43 could be functionally substituted with the yeast prion domain Sup35N, suggesting that amyloid and non-amyloid disease proteins have similar folded domains in healthy cells [18] . This domain participates in a novel type of protein interaction in which the native TDP-43 C-terminus physically interacts with either itself or the folded yeast prion domain Sup35 to form dynamic insoluble aggregates [18] . The aggregation-prone nature of TDP-43 affects its known roles in cellular processes such as subcellular localization, cystic fibrosis transmembrane conductance regulator exon skipping and protein stability [18] . The TDP-43 C-terminus is required for targeting to SGs [19] , suggesting that the intrinsic propensity of the TDP-43 C-terminus to aggregate might be intimately involved in ROS-related pathogenesis. Here we characterize the alterations in TDP-43 multimers in response to an ROS insult by determining how various TDP-43 mutations influence the formation of insoluble TDP-43 polymers in SGs and toxic soluble TDP-43 oligomers. The mutations include misfolded TDP-43 mutants in which the GQN-rich domain fails to fold properly and TDP-43 mutants in which the C-terminus is replaced with the yeast prion Sup35 domain. We determine that TDP-43 multimer assembly is associated with changes in the association between TDP-43 and heat-shock proteins (HSPs), an effect that is influenced by ROS and pharmacological HSP inhibitors. Our study provides a basis for understanding how a disease risk factor affects a disease-causing protein with an intrinsically disordered domain and suggests that a common mechanism could be involved in the pathogenesis of conformational diseases that result from HSP dysregulation. SG targeting and assembly by the prion-like domain (PLD) Upon ROS stimulation, TDP-43 localizes to SGs via its RNA-binding and C-terminal PLDs [10] , [11] , [12] , [19] . We recently demonstrated that the GQN-rich C-terminus of TDP-43 functionally assembles in cells [18] . We were therefore interested in determining whether this intrinsic propensity of the TDP-43 C-terminus to aggregate drove TDP-43 into SGs following an ROS insult, given that the prion-like behaviour of TIA-1 is responsible for SG targeting and assembly [20] . The TDP-43 constructs utilized in this study are depicted in Fig. 1a . After treatment with 1 mM H 2 O 2 , green-fluorescent protein (GFP) fused to full-length TDP-43 (GFP-TDP-43-FL) localized to the cytosolic granules ( Fig. 1a ). The kinetics of TDP-43-positive SG formation was examined via intracellular colocalization with TIAR (red; Supplementary Fig. S1 ). The colocalization of TDP-43 with SGs was determined after treatment with 1 mM H 2 O 2 for 0, 10, 20, 40, 60 or 80 min. The number of TDP-43-positive SGs increases up to 60 min. After 80 min of treatment with 1 mM H 2 O 2 , the TDP-43-positive SGs become larger but decrease in number. TDP-43 mutants that lack the PLD (TDP-43-PLDΔ) or that only contain the PLD (TDP-43-PLD) fail to accumulate in the cytosol ( Fig. 1a ). To validate that a function of the prionogenic domain is to target TDP-43 to SGs, we examined a chimeric TDP-43 mutant (mTDPSupN) in which the PLD of TDP-43 is replaced with the yeast prion domain Sup35N. Similar to GFP-TDP-43-FL, this chimeric protein assembles into the cytosolic granules in response to oxidative stress ( Fig. 1a ). Double staining with the SG marker TIAR (magenta) reveals that the mTDPSupN (green) cytosolic granules localize within SGs ( Fig. 1b , arrow). Conversely, recruitment of the TDP-43 mutant GFP-TDP-43-Q303P after treatment with H 2 O 2 is significantly reduced ( Fig. 1c ). The C-terminus of this mutant is unable to fold properly because of a proline substitution at amino acid 303 (ref. 18 ). The percentage of cells with cytosolic granules containing GFP-TDP-43-FL or GFP-TDP-43-Q303P after H 2 O 2 treatment is presented in the right panel of Fig. 1c . SG-positive cells are defined as cells that contain at least two TDP-43 foci with a minimum diameter of 0.5 μm. The over expression of proteins with functional PLDs, including GFP-TDP-43-FL, GFP-TDP-PLD and GFP-TDPSupN, significantly increase TIAR-positive granule formation upon ROS insult ( Fig. 1d ). A comparison of the ability of the TDP-43 mutants to promote TIAR-containing SG formation is presented in Fig. 1e . The data indicate that the intrinsic aggregation of the TDP-43 C-terminus and the yeast prion domain Sup35N target TDP-43 to SGs in response to oxidative stress. The expression level of the prion-like (prionogenic) domain might determine the number of SGs. 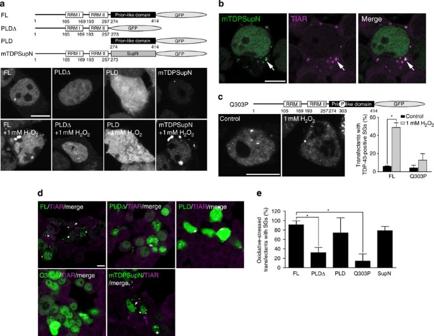Figure 1: The intrinsic propensity to aggregate was required to target TDP-43 to SGs. (a) The cellular localization of TDP-43 variants in the presence or absence of H2O2is depicted. A schematic diagram of the TDP-43 constructs is illustrated at the top. Scale bars: 10 μm. (b) The colocalization of the chimeric mTDPSupN (green) mutant and TIAR (magenta) in SGs was analysed after treatment with 1 mM H2O2. The white colour indicates areas of colocalization (arrows). Scale bars: 10 μm. (c) The cellular distribution of GFP-TDP-43-Q303P in normal and H2O2-treated cells is illustrated. The percentage of SG-positive GFP-TDP-43-FL- or GFP-TDP-43-Q303P-transfected cells was determined, and the statistical analysis is presented in the right panel. The structure of GFP-TDP-43-Q303P is depicted at the top. Scale bars: 10 μm. All the data are presented as the mean±s.d. (n=5). *P<0.05,t-test. (d) SG formation was analysed in cells transfected with GFP-TDP-43-FL, GFP-TDP-43-PLDΔ, GFP-TDP-43-PLD, GFP-TDP-43-Q303P or GFP-TDP-43SupN. Scale bars: 10 μm. (e) A statistical analysis of the oxidative-stressed TDP-43 transfectants that contained SGs was performed. All the data are presented as the mean±s.d. (n=5). *P<0.05,t-test. Figure 1: The intrinsic propensity to aggregate was required to target TDP-43 to SGs. ( a ) The cellular localization of TDP-43 variants in the presence or absence of H 2 O 2 is depicted. A schematic diagram of the TDP-43 constructs is illustrated at the top. Scale bars: 10 μm. ( b ) The colocalization of the chimeric mTDPSupN (green) mutant and TIAR (magenta) in SGs was analysed after treatment with 1 mM H 2 O 2 . The white colour indicates areas of colocalization (arrows). Scale bars: 10 μm. ( c ) The cellular distribution of GFP-TDP-43-Q303P in normal and H 2 O 2 -treated cells is illustrated. The percentage of SG-positive GFP-TDP-43-FL- or GFP-TDP-43-Q303P-transfected cells was determined, and the statistical analysis is presented in the right panel. The structure of GFP-TDP-43-Q303P is depicted at the top. Scale bars: 10 μm. All the data are presented as the mean±s.d. ( n =5). * P <0.05, t -test. ( d ) SG formation was analysed in cells transfected with GFP-TDP-43-FL, GFP-TDP-43-PLDΔ, GFP-TDP-43-PLD, GFP-TDP-43-Q303P or GFP-TDP-43SupN. Scale bars: 10 μm. ( e ) A statistical analysis of the oxidative-stressed TDP-43 transfectants that contained SGs was performed. All the data are presented as the mean±s.d. ( n =5). * P <0.05, t -test. Full size image TDP-43-positive SGs do not cause ROS-induced cell death We conducted live-cell recordings that monitored the stress response in GFP-TDP-43-FL-transfected cells to determine whether TDP-43-positive SGs were involved in ROS-induced cell death ( Fig. 2a ). 293T cells were utilized because they can be efficiently transfected, and TDP-43-positive SGs have been observed in non-neuronal cells from patients. TDP-43-FL-expressing cells were treated with 1 mM H 2 O 2 for 1 h, and cell viability was evaluated by MTT assay after a 24-h recovery period. The MTT assay revealed that GFP-TDP-43-FL expression in transfected cells results in a 5.5-fold decrease in cell viability compared with control cells ( Fig. 2a ). This finding suggests that increased TDP-43 protein levels exacerbate ROS-induced cell death. 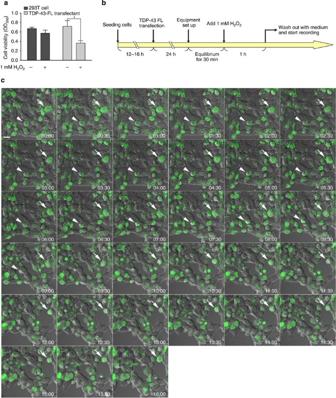Figure 2: Viability of TDP-43-FL-expressing cells after a recovery from H2O2treatment. (a) The reduction in cell viability in response to 1 mM H2O2was enhanced in GFP-TDP-43-FL-overexpressing cells after a 24-h recovery period. All the data are presented as the mean±s.d. (n=3). *P<0.05,t-test. (b) A flow chart of the experimental procedure for live-cell imaging is presented. (c) Images of GFP-mTDP-43-FL-transfected cells were captured using time-lapse microscopy during the recovery period after treatment with 1 mM H2O2. Time-lapse fluorescent images of GFP-mTDP-43-FL-expressing cells were captured every min for 30 min. Cells containing TDP-43-positive SGs (arrowheads) or with diffuse patterns of TDP-43 expression (arrows) are presented as examples. Scale bars: 20 μm. Figure 2: Viability of TDP-43-FL-expressing cells after a recovery from H 2 O 2 treatment. ( a ) The reduction in cell viability in response to 1 mM H 2 O 2 was enhanced in GFP-TDP-43-FL-overexpressing cells after a 24-h recovery period. All the data are presented as the mean±s.d. ( n =3). * P <0.05, t -test. ( b ) A flow chart of the experimental procedure for live-cell imaging is presented. ( c ) Images of GFP-mTDP-43-FL-transfected cells were captured using time-lapse microscopy during the recovery period after treatment with 1 mM H 2 O 2 . Time-lapse fluorescent images of GFP-mTDP-43-FL-expressing cells were captured every min for 30 min. Cells containing TDP-43-positive SGs (arrowheads) or with diffuse patterns of TDP-43 expression (arrows) are presented as examples. Scale bars: 20 μm. Full size image We investigated the role of TDP-43-positive SGs in ROS-induced cell death to determine whether the increase in ROS-induced cell death resulted from increased TDP-43 protein levels and the subsequent formation of TDP-43-positive SGs. We utilized live-cell recordings to monitor the stress levels in GFP-TDP-43-FL-transfected cells during the recovery stage. The experimental procedure utilized to monitor the cells is illustrated in Fig. 2b . We discovered that transfected cells with (arrowhead) or without (arrow) TDP-43-positive SGs exhibit similar cell death rates within a 24-h period ( Fig. 2c ), suggesting that there is no correlation between ROS-induced cell death and the formation of TDP-43-positive SGs ( Supplementary Movie 1 ). Once the recovery began, ~76% of the stressed transfected cells that contained TDP-43-positive SGs continued to accumulate, rather than to disassemble, which contradicts previous studies of fixed cells [10] ( Fig. 2c , arrowhead). ROS induces toxic 130-kDa TDP-43 oligomers at later stages We overexpressed GFP, GFP-TDP-43-FL, GFP-TDPSupN or GFP-TDP-43-Q303P in 293T cells to determine whether ROS-induced cell death is caused by the propensity of the TDP-43 C-terminus to aggregate. After a 24-h recovery from treatment with 0.12 mM H 2 O 2 , cells expressing GFP-TDP-43-FL or GFP-TDPSupN exhibit reduced viability (1.7- and 2.1-fold, respectively) compared with GFP-expressing cells ( Fig. 3a ). Conversely, GFP-TDP-43-Q303P-expressing cells are resistant to H 2 O 2 -mediated cell death ( Fig. 3a ). As the survival increase in the GFP-TDP-43-Q303P-expressing cells likely results from the interference of GFP-TDP-43-Q303P with the self-interactions of the endogenous TDP-43 C-terminus ( Fig. 3a ), we speculated that an additional toxic and self-aggregating TDP-43 species assembles after the H 2 O 2 was removed. Indeed, western blot analysis revealed that after a 24-h recovery from treatment with 0.12 mM H 2 O 2 , a 130-kDa TDP-43 species appears in GFP-TDP-43-FL-expressing cells; there is no increase in this species in GFP-TDP-43-Q303P-expressing cells ( Fig. 3b ). As the disruption of the self-interaction within GFP-TDP-43-Q303P induces protein fragment degradation 3–4 days post transfection [18] , interference experiments with the GFP-TDP-43-Q303P mutant were conducted within 48 h of transfection. 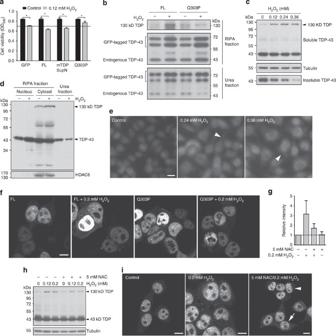Figure 3: GFP-TDP-43-Q303P attenuated ROS-induced cell death and the formation of cytosolic 130-kDa TDP-43 oligomers. (a) GFP-TDP-43-Q303P increased the resistance to H2O2-induced cell death. All the data are presented as the mean±s.d. (n=3). *P<0.05,t-test. (b) GFP-TDP-43-Q303P overexpression blocked the H2O2-induced increase in the formation of 130-kDa TDP-43 oligomers. (c) H2O2increased the levels of 130-kDa TDP-43 and the solubility of TDP-43. (d) H2O2(0.12 mM) increased the cytosolic levels of 130-kDa TDP-43 and increased the nuclear expression of the soluble 43-kDa monomer during a 24-h recovery period after the oxidative insult. (e) Endogenous cytosolic 130-kDa TDP-43 (arrowhead) levels increased in a dose-dependent manner. Scale bars: 10 μm. (f) Cytosolic TDP-43 levels did not increase in GFP-TDP-43-Q303P-expressing cells during a 24-h recovery period after treatment with 0.2 mM H2O2. Scale bars: 10 μm. (g,h) The H2O2-induced formation of 130-kDa TDP-43 was attenuated by NAC. The statistical analysis of the intensity of the 130-kDa TDP-43 bands is presented ing. All the data are presented as the mean±s.d. (n=3). The western blot is illustrated inh. (i) NAC partially suppressed the H2O2-induced increase in endogenous cytosolic TDP-43. The arrowhead indicates NAC-treated cells. The arrow highlights stressed cells that were not inhibited with NAC. Scale bars: 10 μm. Full-sized immunoblots are included inSupplementary Fig. S8. Figure 3: GFP-TDP-43-Q303P attenuated ROS-induced cell death and the formation of cytosolic 130-kDa TDP-43 oligomers. ( a ) GFP-TDP-43-Q303P increased the resistance to H 2 O 2 -induced cell death. All the data are presented as the mean±s.d. ( n =3). * P <0.05, t -test. ( b ) GFP-TDP-43-Q303P overexpression blocked the H 2 O 2 -induced increase in the formation of 130-kDa TDP-43 oligomers. ( c ) H 2 O 2 increased the levels of 130-kDa TDP-43 and the solubility of TDP-43. ( d ) H 2 O 2 (0.12 mM) increased the cytosolic levels of 130-kDa TDP-43 and increased the nuclear expression of the soluble 43-kDa monomer during a 24-h recovery period after the oxidative insult. ( e ) Endogenous cytosolic 130-kDa TDP-43 (arrowhead) levels increased in a dose-dependent manner. Scale bars: 10 μm. ( f ) Cytosolic TDP-43 levels did not increase in GFP-TDP-43-Q303P-expressing cells during a 24-h recovery period after treatment with 0.2 mM H 2 O 2 . Scale bars: 10 μm. ( g , h ) The H 2 O 2 -induced formation of 130-kDa TDP-43 was attenuated by NAC. The statistical analysis of the intensity of the 130-kDa TDP-43 bands is presented in g . All the data are presented as the mean±s.d. ( n =3). The western blot is illustrated in h . ( i ) NAC partially suppressed the H 2 O 2 -induced increase in endogenous cytosolic TDP-43. The arrowhead indicates NAC-treated cells. The arrow highlights stressed cells that were not inhibited with NAC. Scale bars: 10 μm. Full-sized immunoblots are included in Supplementary Fig. S8 . Full size image After a 24-h recovery from H 2 O 2 treatment, we analysed the behaviour of the endogenous 130-kDa TDP-43 species via immunostaining and western blot analysis. The 130-kDa species of TDP-43 accumulated in H 2 O 2 -treated cells in a dose-dependent manner ( Fig. 3c , arrowhead), whereas the concentration of insoluble TDP-43 monomers gradually decreased ( Fig. 3c , bottom panel). Notably, changes in TDP-43 solubility also occurred in GFP-TDP-43-Q303P-expressing cells ( Fig. 3b ), indicating that changes in solubility are not related to ROS-induced cell death ( Fig. 3a,b ). Furthermore, our cell fractionation results suggest that the amount of 130-kDa TDP-43 increased in the cytosol after a 24-h recovery from 0.12 mM H 2 O 2 ( Fig. 3d , arrowhead). Consistent with the fractionation results, cytosolic endogenous TDP-43 translocation occurs in a dose-dependent manner ( Fig. 3e , arrowhead), and the increase in cytosolic TDP-43 negatively correlates with cell viability ( Supplementary Fig. S2 ). Consistent with this observation, GFP-TDP-43-Q303P appeared to be resistant to H 2 O 2 -induced cytosolic translocation ( Fig. 3f ). These data suggest that a cytosolic and toxic oligomer of TDP-43 was associated with ROS-induced cell death. The effects of ROS on the assembly of the 130-kDa TDP-43 oligomers were confirmed using N-acetylcysteine (NAC), an ROS scavenger ( Fig. 3g,h ). Pretreating cells with NAC attenuated the H 2 O 2 -induced accumulation of 130-kDa TDP-43 ( Fig. 3g,h ), increased cell death ( Supplementary Fig. S3 ) and partially inhibited the H 2 O 2 -induced cytosolic translocation of endogenous TDP-43 in a subset of cells ( Fig. 3i , arrowhead). The arrow in Fig. 3i indicates stressed cells without NAC inhibition. Previous studies have reported that increased cytosolic TDP-43 is related to the degradation of the TDP-43 C-terminus and the formation of pathological inclusions. However, ROS induces the assembly of cytosolic TDP-43 into toxic and soluble 130-kDa oligomers. ROS-induced TDP-43 oligomers regulate oxidative stress We next determined whether the ROS-induced formation of TDP-43 oligomers regulates oxidation-sensitive proteins, therefore disrupting normal physiological processes. Several oxidation-related molecules have been identified, including oxidation-sensitive proteins in metabolic pathways and signal transducers within the PI3K-AKT pathway. In addition, HSPs and NAD + regulatory factors, such as PARP and SIRT1, are involved in oxidative stress [21] . The western blot analysis indicated that GFP-TDP-43-Q303P expression suppressed the oxidative response in particular pathways, including decreasing AKT phosphorylation and reducing the levels of pro-caspase 3, PARP, PGC-1α and HSPs ( Fig. 4a,c ). After H 2 O 2 treatment, GFP-TDP-43-FL and GFP-TDP-43-Q303P downregulated the expression of AKT, SIRT1 and HDAC6. However, AKT, SIRT1 and HDAC6 are not downregulated in GFP-expressing cells ( Fig. 4b ). These data imply that the regulation of these three proteins in stressed cells is dependent on the RNA-binding domain of TDP-43. HSP27 expression was downregulated by three different constructs ( Fig. 4d ). HSP90 and HSP70 are specifically upregulated in GFP-TDP-43-FL-expressing cells; this may result from the ROS-induced formation of the 130-kDa TDP-43 species ( Supplementary Fig. S4 ). The expression of the oxidation-related protein HSP32 increases in cells expressing either GFP-TDP-43-FL or GFP-TDP-43-Q303P ( Supplementary Fig. S4 ). Along with the data in Fig. 3a , these data suggest that the deficiencies in ROS-induced alterations to p-AKT, PARP, PGC-1α, pro-caspase 3 and HSP levels might be related to the increased resistance to cell death in GFP-TDP-43-Q303P-overexpressing cells ( Fig. 4a,c ). Therefore, the 130-kDa TDP-43 oligomers act as an upstream regulator of oxidative stress. 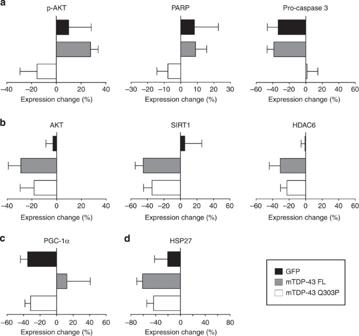Figure 4: Redox-sensitive protein expression profiles in TDP-43-expressing cells treated with H2O2. (a) Western blots illustrate the effects of H2O2in GFP-, GFP-TDP-43-FL- or GFP-TDP-43-Q303P-expressing cells. Treating transfected cells with 0.2 mM H2O2for 30 min, followed by a 24-h recovery period, significantly increased p-AKT and PARP levels and decreased pro-caspase 3 levels in GFP- and TDP-43-FL-expressing cells but not in GFP-TDP-43-Q303P-expressing cells. (b) After H2O2treatment, AKT, SIRT1 and HDAC6 expression was downregulated in GFP-TDP-43-FL- and GFP-TDP-43-Q303P-expressing cells but not in GFP-expressing cells. (c) Treatment with 0.2 mM H2O2increased PGC-1α expression in TDP-43-FL-expressing cells. (d) Treatment with 0.2 mM H2O2decreased HSP27 expression in all the transfected cells. All the data are presented as the mean±s.d. (n=3). Figure 4: Redox-sensitive protein expression profiles in TDP-43-expressing cells treated with H 2 O 2 . ( a ) Western blots illustrate the effects of H 2 O 2 in GFP-, GFP-TDP-43-FL- or GFP-TDP-43-Q303P-expressing cells. Treating transfected cells with 0.2 mM H 2 O 2 for 30 min, followed by a 24-h recovery period, significantly increased p-AKT and PARP levels and decreased pro-caspase 3 levels in GFP- and TDP-43-FL-expressing cells but not in GFP-TDP-43-Q303P-expressing cells. ( b ) After H 2 O 2 treatment, AKT, SIRT1 and HDAC6 expression was downregulated in GFP-TDP-43-FL- and GFP-TDP-43-Q303P-expressing cells but not in GFP-expressing cells. ( c ) Treatment with 0.2 mM H 2 O 2 increased PGC-1α expression in TDP-43-FL-expressing cells. ( d ) Treatment with 0.2 mM H 2 O 2 decreased HSP27 expression in all the transfected cells. All the data are presented as the mean±s.d. ( n =3). Full size image HSPs regulate the functional assembly of TDP-43 multimers Previous studies have suggested that several small HSPs and other HSPs, particularly HSP90, associate with TDP-43 (refs 22 , 23 ). As HSP expression, in particular the downregulation of HSP27, is dynamically regulated by the presence or absence of excess ROS ( Fig. 5a ), we investigated whether the assembly of insoluble TDP-43 multimers (aggregates) was influenced by HSP activity ( Fig. 5b–f ). We validated the role of HSPs in ROS-induced TDP-43 multimer assembly by treating cells with 17-AAG to interfere with HSP levels. 17-AAG inhibits HSP90 activity but activates HSF-1, HSP27 and HSP70. Cells were pretreated with 180 nM 17-AAG for 24 h, which suppressed ROS-induced TDP-43 multimer formation in the insoluble fraction ( Fig. 5b ). Consistent with this analysis, 17-AAG inhibits the targeting of TDP-43-FL and the ALS-associated mutant TDP-43-R361S to SGs in response to H 2 O 2 treatment ( Fig. 5c,d ). We confirmed via western blot that 17-AAG inhibits ROS-induced HSP90 degradation, increases HSP70 expression and restores HSP27 expression under conditions of oxidative stress ( Fig. 5e,f ). 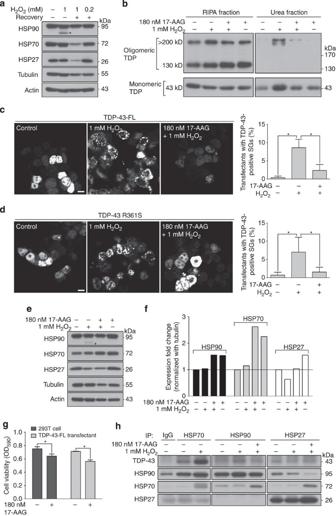Figure 5: 17-AAG inhibited the ROS-induced formation of insoluble TDP-43 multimers and SGs. (a) The HSP expression profiles after a 24-h recovery period from treatment with or without 0.2 or 1 mM H2O2were validated using western blot. Notably, the ROS insult resulted in a degraded HSP90 fragment (asterisk). (b) 17-AAG inhibited the H2O2-induced polymerization of TDP-43 and shift of TDP-43 into the insoluble fraction, as evidenced using western blot. (c) 17-AAG inhibited the H2O2-induced targeting of GFP-TDP-43-FL to SGs. The number of cells containing TDP-43-positive SGs was analysed. Scale bars: 10 μm. All the data are presented as the mean±s.d. (n=3). *P<0.05,t-test. (d) 17-AAG inhibited the H2O2-induced targeting of GFP-TDP-43-R361S to SGs. The number of cells containing TDP-43-positive SGs was analysed. Scale bars: 10 μm. All the data are presented as the mean±s.d. (n=3). *P<0.05,t-test. (e) A western blot analysis was performed to determine the HSP expression profiles in cells pretreated with 180 nM 17-AAG and then treated with or without 1 mM H2O2. *degraded HSP90 fragment. (f) The HSP expression intensity inewas analysed. (g) MTT cell viability assays were performed on cells pretreated or not with 17-AAG. All the data are presented as the mean±s.d. (n=3). *P<0.05,t-test. (h) Co-IPs of TDP-43 and HSPs were performed in cells pretreated with 17-AAG and treated with or without 1 mM H2O2. Full-sized immunoblots are included inSupplementary Fig. S8. Figure 5: 17-AAG inhibited the ROS-induced formation of insoluble TDP-43 multimers and SGs. ( a ) The HSP expression profiles after a 24-h recovery period from treatment with or without 0.2 or 1 mM H 2 O 2 were validated using western blot. Notably, the ROS insult resulted in a degraded HSP90 fragment (asterisk). ( b ) 17-AAG inhibited the H 2 O 2 -induced polymerization of TDP-43 and shift of TDP-43 into the insoluble fraction, as evidenced using western blot. ( c ) 17-AAG inhibited the H 2 O 2 -induced targeting of GFP-TDP-43-FL to SGs. The number of cells containing TDP-43-positive SGs was analysed. Scale bars: 10 μm. All the data are presented as the mean±s.d. ( n =3). * P <0.05, t -test. ( d ) 17-AAG inhibited the H 2 O 2 -induced targeting of GFP-TDP-43-R361S to SGs. The number of cells containing TDP-43-positive SGs was analysed. Scale bars: 10 μm. All the data are presented as the mean±s.d. ( n =3). * P <0.05, t -test. ( e ) A western blot analysis was performed to determine the HSP expression profiles in cells pretreated with 180 nM 17-AAG and then treated with or without 1 mM H 2 O 2 . *degraded HSP90 fragment. ( f ) The HSP expression intensity in e was analysed. ( g ) MTT cell viability assays were performed on cells pretreated or not with 17-AAG. All the data are presented as the mean±s.d. ( n =3). * P <0.05, t -test. ( h ) Co-IPs of TDP-43 and HSPs were performed in cells pretreated with 17-AAG and treated with or without 1 mM H 2 O 2 . Full-sized immunoblots are included in Supplementary Fig. S8 . Full size image 17-AAG-treated cells express increased levels of 130-kDa TDP-43 oligomers in the soluble fraction ( Fig. 5b ) and exhibit reduced cell viability ( Fig. 5g and Supplementary Fig. S5 ). This is consistent with our aforementioned findings ( Fig. 3 ), specifically that soluble 130-kDa TDP-43 oligomers are toxic. Notably, pretreating stressed cells with 17-AAG fails to induce the formation of insoluble TDP-43 polymers ( Fig. 5b ), suggesting that ROS does not freely oxidize TDP-43. Therefore, we speculate that ROS-induced stress alters the expression of TDP-43-associated HSPs, resulting in the disassociation and repartitioning of TDP-43-HSP complexes, the reassembly of TDP-43 multimers and the oxidation of TDP-43. To test our hypothesis, we investigated the physical interaction between TDP-43 and HSPs in the presence or absence of H 2 O 2 and 17-AAG. After H 2 O 2 treatment, the interaction between TDP-43 and HSP90 or HSP70 increases; however, the association between TDP-43 and HSP27 decreases. Pretreating cells with 17-AAG before the ROS insult slightly rescues the association between TDP-43 and HSP27 but reduces the interaction between TDP-43 and HSP90 ( Fig. 5h ). Together with the results in Fig. 3 , these data suggest that the disassociation of TDP-43 from HSP27 might contribute to the generation of insoluble TDP-43 polymers immediately after an ROS insult. However, reduced HSP90 activity might promote the subsequent formation of 130-kDa TDP-43 oligomers because of the stress caused by HSP90 degradation. We performed independent experiments in which we directly interfered with the HSP network balance to ascertain the effects of TDP-43-associated HSPs on the intrinsic aggregation of TDP-43. We inhibited heat-shock-induced HSP expression by pretreating cells with the HSF-1 inhibitor KRIBB11. Subsequently, we evaluated TDP-43 multimer assembly by monitoring the formation of TDP-43 aggregates. After heat shock, TDP-43 aggregates are formed in KRIBB11-pretreated cells but not in untreated control cells ( Supplementary Fig. S6a ). The percentage of cells that contained TDP-43 aggregates increased in a dose-dependent manner ( Supplementary Fig. S6b ). The KRIBB11-mediated inhibition of HSF-1 activity was confirmed ( Supplementary Fig. S6c ), and the expression levels of the corresponding HSPs were validated ( Supplementary Fig. S6d ). Notably, HSP27, but not the other HSPs, significantly reduce in KRIBB11-treated cells. All these results suggest that the aggregation-prone nature of TDP-43 is tightly correlated with the cellular TDP-43-associated HSP content. 17-AAG alleviates pathological TDP-43 aggregation 17-AAG treatment also reduces the levels of pathological misfolded TDP-43 C-terminus aggregates (GFP-TDP-43-IIPLD) in a dose-dependent manner within 24 h ( Fig. 6a ) [18] . The GFP-TDP-43-IIPLD structure, which mimics the pathological degraded fragment, is illustrated at the top of Fig. 6a . The statistical analysis of the pathological aggregates is presented in Fig. 6b , and western blotting was utilized to confirm these results ( Fig. 6c,d ). A significant increase in GFP-TDP-43-IIPLD solubility was observed in 17-AAG-treated cells ( Fig. 6c ). The solubility ratio is presented in Fig. 6d . The effects of 17-AAG on HSP expression levels were validated ( Fig. 6c and Supplementary Fig. S7 ). 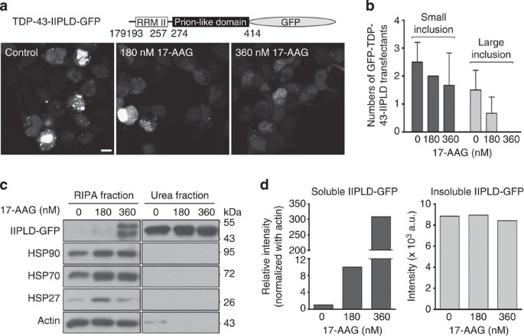Figure 6: 17-AAG reduced the number of pathological TDP-43 aggregates. (a) 17-AAG reduced the number of pathological aggregates that contained TDP-43 C-terminal fragments. The GFP-TDP-43-IIPLD structure that mimics the pathological degraded fragment is illustrated at the top. (b) The number of cells that contained small (<5 μm diameter) or large (>5 μm diameter) TDP-43 aggregates is presented. Scale bars: 10 μm. All the data are presented as the mean±s.d. (n=3). (c) Western blotting was utilized to illustrate the effects of 17-AAG on GFP-TDP-43-IIPLD solubility. (d) The relative intensity of GFP-TDP-43-IIPLD expression incwas analysed. Full-sized immunoblots are included inSupplementary Fig. S8. Figure 6: 17-AAG reduced the number of pathological TDP-43 aggregates. ( a ) 17-AAG reduced the number of pathological aggregates that contained TDP-43 C-terminal fragments. The GFP-TDP-43-IIPLD structure that mimics the pathological degraded fragment is illustrated at the top. ( b ) The number of cells that contained small (<5 μm diameter) or large (>5 μm diameter) TDP-43 aggregates is presented. Scale bars: 10 μm. All the data are presented as the mean±s.d. ( n =3). ( c ) Western blotting was utilized to illustrate the effects of 17-AAG on GFP-TDP-43-IIPLD solubility. ( d ) The relative intensity of GFP-TDP-43-IIPLD expression in c was analysed. Full-sized immunoblots are included in Supplementary Fig. S8 . Full size image The western blots in Fig. 5b were performed under reducing conditions, with dithiothreitol in the sample loading buffer. This excluded the possibility of intra- and interdisulfide crosslinking by oxidization, which is the major mechanism for generating ROS-induced insoluble TDP-43 polymers [10] . In the present study, we suggested that ROS altered the reassembly of TDP-43 multimers by modulating TDP-43-associated HSPs ( Fig. 7 ). Immediately after an ROS insult, TDP-43 was targeted to SGs and assembled into insoluble TDP-43 polymers. During later stages, the levels of toxic and soluble 130-kDa TDP-43 significantly increased in the cytosol. Interestingly, an ~130-kDa version of TDP-43 has been identified in the brains of patients with FTLD-U [10] . These soluble TDP-43 oligomers, which form because of a propensity towards intrinsic aggregation, regulate crucial molecules involved in oxidative signalling, particularly PARP and HSPs. Although increased levels of cytosolic TDP-43 has been previously reported, we did not observe any TDP-43 pathological aggregates in stressed cells after H 2 O 2 treatment. The data suggested that oxidative stress was not the pathogenic factor that was directly responsible for the TDP-43 cleavage that has been observed in patients with FTLD-U or ALS. Nevertheless, the increase in cytosolic 130-kDa TDP-43 oligomers that resulted from excess ROS led to cell death; these oligomers might be the major contributor to the pathogenesis of these particular diseases during the early pre-symptom stage. We propose that this pre-existing physiological imbalance could promote neuronal death at later stages, when secondary risk factors appear ( Fig. 7 ) [24] . 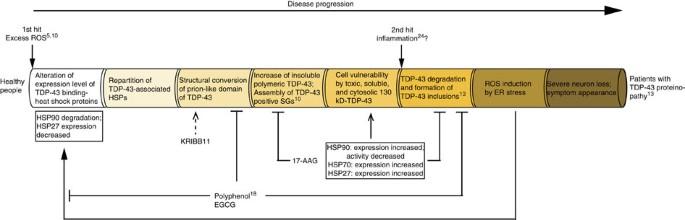Figure 7: Proposed timeline for the progression of ROS-related molecular pathology in TDP-43-related proteinopathies. The proposed model illustrates the sequential changes in the physical and chemical properties of TDP-43 polymers that occur in the presence of excess ROS and includes a novel 130-kDa TDP-43 oligomer that is involved in oxidative stress transduction. In healthy cells, the native monomeric TDP-43 C-terminus physically interacts with itself or with other prion-like domains to form functional aggregates. Elevated intracellular ROS levels typically occur during aging and in the early stages of neurodegeneration. In the presence of excess ROS, the HSP expression profiles are immediately altered in response to the repartitioning of TDP-43-associated HSPs, and TDP-43 is targeted to SGs and assembles into insoluble TDP-43 polymers. At later stages, the levels of toxic soluble 130-kDa TDP-43 oligomers significantly increases and affects redox signalling and cell viability. The ROS-induced sequential reassembly of TDP-43 polymers is the first indication of a TDP-43 proteinopathy. A second risk factor, such as inflammation, can cause further degradation of the TDP-43 C-terminus. The degraded TDP-43 C-terminal fragments form pathological inclusions. These TDP-43 inclusions induce ER stress following ROS generation, leading to massive neuron death and brain atrophy. Compounds that function at different stages in TDP-43 proteinopathies are indicated. Figure 7: Proposed timeline for the progression of ROS-related molecular pathology in TDP-43-related proteinopathies. The proposed model illustrates the sequential changes in the physical and chemical properties of TDP-43 polymers that occur in the presence of excess ROS and includes a novel 130-kDa TDP-43 oligomer that is involved in oxidative stress transduction. In healthy cells, the native monomeric TDP-43 C-terminus physically interacts with itself or with other prion-like domains to form functional aggregates. Elevated intracellular ROS levels typically occur during aging and in the early stages of neurodegeneration. In the presence of excess ROS, the HSP expression profiles are immediately altered in response to the repartitioning of TDP-43-associated HSPs, and TDP-43 is targeted to SGs and assembles into insoluble TDP-43 polymers. At later stages, the levels of toxic soluble 130-kDa TDP-43 oligomers significantly increases and affects redox signalling and cell viability. The ROS-induced sequential reassembly of TDP-43 polymers is the first indication of a TDP-43 proteinopathy. A second risk factor, such as inflammation, can cause further degradation of the TDP-43 C-terminus. The degraded TDP-43 C-terminal fragments form pathological inclusions. These TDP-43 inclusions induce ER stress following ROS generation, leading to massive neuron death and brain atrophy. Compounds that function at different stages in TDP-43 proteinopathies are indicated. Full size image In our study, the HSP90 inhibitor 17-AAG inhibited ROS-induced insoluble TDP-43 polymerization and disassembled the pathological TDP-43 aggregates ( Figs 5b-d , 6 ). Although 17-AAG eventually increased the levels of toxic 130-kDa TDP-43, we did not observe a significant increase in toxic 130-kDa TDP-43 levels within 12 h of 17-AAG treatment; rather, during this time period, we observed the disassembly of pathological inclusions. This observation led us to propose 17-AAG as a potential candidate for therapeutic use in patients with TDP-43 inclusions. A safer approach might be to combine 17-AAG with stabilizers of native TDP-43. A previous study demonstrated that oral 17-AAG administration suppressed polyglutamine-induced inclusions and neurodegeneration in fly models of SCA and Huntington’s disease by activating HSF-1 and multimolecular chaperones [25] . Furthermore, SOD G93A mice, which express an ALS-associated SOD1 mutation, exhibited significant functional improvements in their hind limb muscles and motor neurons and a 22% increase in lifespan after treatment with arimoclomol, a co-inducer of HSP70 and HSP90 [26] . Consistent with the pharmacological studies, the effects of HSPs on the yeast prion conformational change, propagation and formation under stress conditions, such as heat shock, have been characterized [27] , [28] , [29] , [30] , [31] , [32] . These studies suggested that HSPs could be effective against various conformational diseases. Factors that affect HSPs could be utilized to regulate intrinsically disordered protein conformations, active or inactive biological processes and pathogenesis. The HSP expression profiles were exquisitely sensitive to physiological perturbations, such as oxidative stress ( Fig. 5a ). TDP-43 physically associated with numerous HSPs at different subcellular locations, suggesting that individual HSP-TDP-43 complexes might participate in distinct biological processes. Therefore, reducing the levels of a particular TDP-43-associated HSP might shift the intrinsically disordered region into a different or misfolded conformation or lead to degradation. Compared with other cell types, neurons have an ~10-fold greater sensitivity to oxidative stress, suggesting that reducing oxidative-induced damage is critical for the prevention of neurodegenerative disease ( Fig. 7 ). Excepting the use of antioxidants, an alternative approach to preventing neurodegenerative disease is to increase neuronal cell tolerance to oxidative stress by upregulating the expression of appropriate HSPs. A promising approach to redirecting the pathological progression of intrinsic aggregation is the targeting of TDP-43-associated molecular chaperones (for example, via 17-AAG treatment). The maintenance of functional intrinsically disordered proteins throughout a lifespan is a prominent issue that needs to be addressed. Cell culture and drug treatment HEK293T (CRL11268; ATCC, Manassas, VA, USA) cells were grown in Dulbecco’s modified Eagle's medium (DMEM)/F12 supplemented with 10% fetal bovine serum and 1% penicillin/streptomycin. HEK293T cells were transfected via the calcium phosphate protocol as per the manufacturer’s instructions. Full-length TDP-43 cDNA was amplified from pools of mouse brain cDNA and cloned into pEGFP-N3 (Clontech, Mountain View, CA, USA). GFP-TDP-43-FL was utilized to generate GFP-tagged TDP-43 variants. All the primers utilized for plasmid construction are listed in Table 1 (ref. 18 ). HEK293T cells (1 × 10 5 ) were seeded into six-well plates and incubated overnight in a 37 °C incubator with 5% CO 2 . For the H 2 O 2 -induced oxidative stress studies, the cells were pretreated with the indicated concentration of H 2 O 2 (0.1, 0.2 or 0.4 mM) for 30 min or with 1 mM H 2 O 2 for 1 h. Fresh medium was added, and the cells were incubated at 37 °C for 24 h. To determine the effect of 17-AAG on H 2 O 2 -induced cell viability, the cells were pretreated with or without 180 or 360 nM 17-AAG for 24 h prior to treatment with 1 mM H 2 O 2 for 1 h. In the heat-shock experiment, cells expressing GFP-TDP-43-FL were pretreated with KRIBB11 at the indicated concentration at 37 °C for 1 h. The cells were subsequently incubated at 42 °C for 30 min, followed by a recovery at 37 °C for 1 h. Table 1 Primers used for plasmid construction of GFP-tagged mTDP-43 variants. Full size table Reagents and antibodies Hydrogen peroxide was purchased from Merck (Whitehouse Station, NJ, USA). 17-AAG was purchased from Sigma-Aldrich (St. Louis, MO, USA) and dissolved in dimethyl sulfoxide. Primary antibodies against p-AKT (Ser473, 9271S, 1:2,000 dilution), AKT (9272, 1:2,000), PARP (9542S, 1:2,000), caspase 3 (9668S, 1:2,000), PGC-1α (2178S, 1:2,000), HSP27 (2402S, 1:2,000) and β-tubulin (2146S, 1:15,000) were purchased from Cell Signalling Technology (Beverly, MA, USA). A primary antibody against TDP-43 (12892-1-AP, 1:10,000) was purchased from Proteintech (Chicago, IL, USA). A primary antibody against HSP90 (610419, 1:2,000) was purchased from BD (Franklin Lakes, NJ, USA). A primary antibody against SIRT1 (05-1243, 1:2,000) was purchased from Millipore (Billerica, MA, USA). Primary antibodies against HDAC6 (ab47181, 1:2,000) and HSP70 (ab2787, 1:2,000) were purchased from Abcam (Cambridge, MA, USA). A primary antibody against HSP32 (OSA-111, 1:2,000) was purchased from Assay designs (Farmingdale, NY, USA). Cell viability assay HEK293T cells (2.5 × 10 4 ) were seeded into 24-well plates and incubated in DMEM/F12 containing serum at 37 °C and 5% CO 2 . After an overnight incubation, the cells were transfected with GFP-tagged mTDP-43-FL. After a post-transfection period (12 h), the cells were treated with the indicated concentration of H 2 O 2 for 30 min or 1 h. The cells were then incubated for an additional 24 h. The MTT assays were performed according to the manufacturer’s instructions (Promega, Madison, WI, USA). Fluorescence was measured at 590 nm. Three independent experiments were performed. TDP-43 solubility assay Cells that had been transfected with or without GFP-TDP-43-FL or GFP-TDP-43-Q303P were lysed in RIPA buffer (50 mM Tris, 150 mM NaCl, 1 mM EDTA and 1% NP-40; pH 7.4), and the lysates were fractionated using centrifugation at 16,000 g for 5 min at 4 °C. The insoluble pellets were dissolved in 8 M urea/50 mM Tris (pH 8.0). TDP-43 was identified via western blotting using a polyclonal TDP-43 antibody. Image acquisition The cells were plated on cover slips. Treated or untreated cells were fixed with 3.7% paraformaldehyde in phosphate-buffered saline at room temperature (RT) for 10 min, according to an immunostaining protocol [33] . The fixed cells were incubated with an antibody against TDP-43 (1:500 dilution) or TIAR (610352, 1:500 dilution) (BD) at 4 °C overnight followed by an incubation with a secondary antibody conjugated to a fluorescent dye at RT for 1 h. The cover slips were mounted with mounting medium (Sigma-Aldrich), and the fluorescent images were acquired with a fluorescent microscope (IX71; Olympus, Center Valley, PA, USA) or a laser confocal microscope (LSM710 META or LSM510 META NLO; Zeiss, Thornwood, NY, USA). Live-cell imaging HEK293T cells were plated on cover slides and transfected with GFP-TDP-43-FL. Transfected cells were maintained at 37 °C on a heated stage with 5% CO 2 . The detailed experimental procedure is illustrated in Fig. 2b . All the 16-bit images were obtained with a Zeiss LSM710, and a 40/1.4 NA lens was utilized for these experiments. The laser spectrum was set to a wavelength of 488 nm and an intensity <1.25% of the total power (25%). The total recording time was 24 h. Statistical analysis The statistical significance was calculated using analysis of variance ( t -test). Differences between the groups were considered to be significant if the P -value was <0.05. How to cite this article: Chang, H.-Y. et al . Heat-shock protein dysregulation is associated with functional and pathological TDP-43 aggregation. Nat. Commun. 4:2757 doi: 10.1038/ncomms3757 (2013).